Super-resolution photoacoustic imaging through a scattering wall The use of wavefront shaping to compensate for scattering has brought a renewed interest as a potential solution to imaging through scattering walls. A key to the practicality of any imaging through scattering technique is the capability to focus light without direct access behind the scattering wall. Here we address this problem using photoacoustic feedback for wavefront optimization. By combining the spatially non-uniform sensitivity of the ultrasound transducer to the generated photoacoustic waves with an evolutionary competition among optical modes, the speckle field develops a single, high intensity focus significantly smaller than the acoustic focus used for feedback. Notably, this method is not limited by the size of the absorber to form a sub-acoustic optical focus. We demonstrate imaging behind a scattering medium using two different imaging modalities with up to ten times improvement in signal-to-noise ratio and five to six times sub-acoustic resolution. Imaging through opaque, highly scattering walls is a long sought after capability with potential applications in a variety of fields [1] . Recent advances in wavefront shaping have made this task a possibility [2] , [3] , [4] , [5] , [6] , [7] , [8] , [9] , [10] , [11] , [12] . By precompensating the optical wavefront, the light propagation can be controlled through and beyond scattering materials [2] , [3] , [13] , [14] . Most existing techniques, however, are limited by their need to generate feedback from behind or inside a scatterer with direct invasive access. Several recent techniques have overcome this limitation using acoustic waves, either with an ultrasound guide-star [15] or a photoacoustic feedback [16] , [17] , [18] . Two modifications of the ultrasound guide-star method have allowed for the creation of an optical focus smaller than the acoustic spot size [19] , [20] . Si et al . [19] frequency modulated diffuse light with a focused ultrasound transducer and then time reversed the encoded light using optical phase conjugation. Through iterative time reversal, a convergence of the light to the central region of the ultrasound focal volume where the modulation is the strongest was observed, resulting in an increase in the optical intensity in a sub-acoustic focal region. Alternatively, the time reversal of variance encoded light approach was also shown to break the acoustic resolution barrier by isolating the spatial location of optical speckles within the ultrasound focus. While both of these techniques are promising for deep fluorescence imaging in scattering materials, their inherent low signal-to-noise ratio (SNR) could limit implementation. Photoacoustics, where acoustic waves are generated from optical absorption and subsequent thermal expansion, has also been used for wavefront optimization [16] , [17] , [18] . In this case, the pressure of the generated acoustic wave is proportional to the light fluence. Hence, the detected photoacoustic wave provides a measure of the local light intensity, facilitating feedback and allowing for wavefront optimization. Only lately has imaging through scattering media been demonstrated using photoacoustic feedback [18] . Without optical focusing, photoacoustic resolution is determined by the ultrasound frequency and numerical aperture of the transducer. Considering a focused ultrasound transducer, uniform optical absorption excites acoustic waves throughout the focal region. However, as shown below, introduction of a scattering material creates a non-uniform optical field with separate and distinct speckle grains. This, in turn, generates spatially varying photoacoustic sources that are integrated over the transducer focus to yield the photoacoustic response. Previous work using photoacoustic feedback with wavefront shaping has assumed that this feedback would create an optical focus limited by the size of the acoustic focus [16] , [17] . With this assumption, a smaller optical focus could be created only when optimizing with sub-acoustic sized absorbers as targets [17] . Here, we demonstrate that by introducing a scattering element into the optical illumination path both SNR and resolution can be improved with wavefront shaping, enabling super-resolution imaging. To accomplish this, the optical intensity of the speckle field within the transducer focus is redistributed to create a single overpowering speckle grain smaller than the ultrasound transducer focus. Thus, the speckle grain acts as an optical focus and improves both photoacoustic emission and resolution over the traditional photoacoustic imaging modality. Such capabilities enable superb three-dimensional imaging of complex biological structures. Simulation of wavefront optimization Optimizing the optical intensity distribution within the ultrasound transducer focal region presents significant challenges because several speckles are present ( Fig. 1a,c ). If multiple optical speckles contribute to the photoacoustic response with equal weighting, the feedback signal uniformly mixes the information coming from individual speckle and does not lead to focus optimization. However, the ultrasound transducer focal region does not detect acoustic waves uniformly. Instead, a focused ultrasound transducer displays a Gaussian spatial sensitivity, which essentially weights the photoacoustic response generated by the optical speckle; giving higher weighting to signals generated closer to the centre ( Fig. 1c ). By preferentially weighting the photoacoustic response produced by a single optical speckle, the spatially non-uniform photoacoustic feedback localizes the optical intensity over an area that is smaller than the acoustic focus ( Fig. 1b,c ). 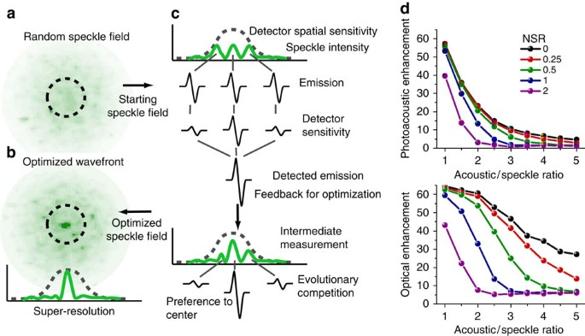Figure 1: Optical focus creation with photoacoustic feedback: illustration and simulation. (a) The transducer focal region (dotted circle) illuminated with a speckle field (b) The optimized speckle field with a sub-acoustic optical focus. (c) Profile of speckle grains and the detector spatial sensitivity. Each photoacoustic emission from the speckle grains is weighted by the Gaussian spatial sensitivity of the acoustic transducer. These emissions coherently combine to provide the photoacoustic feedback signal. During wavefront optimization with the photoacoustic feedback an optical focus forms at the centre of the acoustic transducer due to the weight preference. (d) Simulation results of the photoacoustic and optical enhancements achieved after genetic algorithm optimization with various acoustic focus to speckle size ratios and noise-to-signal ratios. Figure 1: Optical focus creation with photoacoustic feedback: illustration and simulation. ( a ) The transducer focal region (dotted circle) illuminated with a speckle field ( b ) The optimized speckle field with a sub-acoustic optical focus. ( c ) Profile of speckle grains and the detector spatial sensitivity. Each photoacoustic emission from the speckle grains is weighted by the Gaussian spatial sensitivity of the acoustic transducer. These emissions coherently combine to provide the photoacoustic feedback signal. During wavefront optimization with the photoacoustic feedback an optical focus forms at the centre of the acoustic transducer due to the weight preference. ( d ) Simulation results of the photoacoustic and optical enhancements achieved after genetic algorithm optimization with various acoustic focus to speckle size ratios and noise-to-signal ratios. Full size image Simulations of the wavefront optimization elucidate the mechanism by which a spatially non-uniform sensitivity produces a tight optical focus when multiple modes participate in the feedback (see Supplementary Methods for details). Here we use an evolutionary algorithm [21] that creates competition among optical modes within the acoustic focus. The number of modes, determined by the acoustic spot to optical speckle size ratio, and noise (noted as noise-to-signal ratio: NSR) are varied and the optimized photoacoustic signal and optical field analyzed. The wavefront optimization feedback uses an equivalent photoacoustic signal by integrating the total weighted light fluence throughout the acoustic focus. The signal improvement is assessed by photoacoustic enhancement, defined as the optimized photoacoustic signal divided by the mean of the photoacoustic signals of the initial population in the genetic algorithm [21] . In contrast, the optical enhancement evaluates the improvement in the maximum intensity of an individual speckle output mode as the ratio between its intensity and the initial average intensity. Interestingly, the optical enhancement outperforms the photoacoustic enhancement as the number of modes is increased ( Fig. 1d ). The photoacoustic enhancement is integrated over the acoustic focal area while the optical enhancement is not. This indicates the optical energy localizes to an area smaller than the acoustic focus, creating an optical focus regardless of the small speckle size compared with the acoustic feedback. Furthermore, the optimized optical field most likely positions the enhanced speckle at the centre of the acoustic focus (see Supplementary Fig. 1 ). Thus, despite optimizing the wavefront based on feedback from multiple optical speckle modes within the acoustic focus, the light localizes to a single speckle, creating an optical focus. Experimental sub-acoustic focus creation We experimentally demonstrate the ability to localize a scattered light field to a sub-acoustic focus via photoacoustic feedback using the system shown in Fig. 2a . The position of the transducer is not critical in these experiments, so long as the acoustic waves can effectively propagate from the focal point to the transducer face. For this demonstration a 50-μm diameter black alpaca hair that overfills the transducer focal region is selected for photoacoustic feedback. The laser pulse passes through a diffuser, producing the optical intensity pattern at the transducer focal plane shown in Fig. 2b (see Methods section). The optical speckle size, measured through autocorrelation of this image, is ∼ 13 μm. 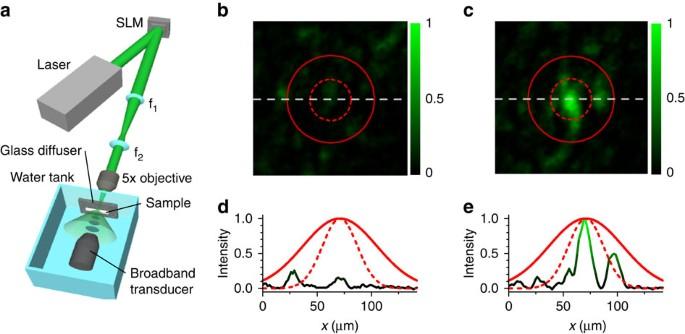Figure 2: Experimental sub-acoustic focus creation. (a) Experimental set-up. (b) The optical speckle field at the photoacoustic imaging plane without the optimized wavefront. (c) The sub-acoustic optical focus generated by the optimized wavefront. The red circles show the approximate filtered transducer focal region (80 MHz, −6 dB, dashed line) and focal spot size at the frequency peak of the detected photoacoustic response (50 MHz, −6 dB, solid line). (d,e) Cross sections of the approximate transducer focal regions (red) and the corresponding optical intensity distribution (black). Figure 2: Experimental sub-acoustic focus creation. ( a ) Experimental set-up. ( b ) The optical speckle field at the photoacoustic imaging plane without the optimized wavefront. ( c ) The sub-acoustic optical focus generated by the optimized wavefront. The red circles show the approximate filtered transducer focal region (80 MHz, −6 dB, dashed line) and focal spot size at the frequency peak of the detected photoacoustic response (50 MHz, −6 dB, solid line). ( d , e ) Cross sections of the approximate transducer focal regions (red) and the corresponding optical intensity distribution (black). Full size image The high bandwidth acoustic transducer provides a wide range of frequency feedback. Because the transducer focal size inversely relates to frequency, the photoacoustic optimization signal is high-pass filtered, effectively limiting the acoustic focal diameter (−6 dB) to 38 μm, as shown by the dashed line in Fig. 2d . After genetic algorithm optimization of the optical wavefront through phase modulation with the spatial light modulator (SLM), the photoacoustic signal is enhanced by 8.5. The optimization creates a 13 μm (Full width at half maximum (FWHM)) focused spot ( Fig. 2c,e ), with an optical enhancement of 24, or three times the photoacoustic enhancement. As predicted, a small, single speckle optical focus is created despite integrating many speckle output modes within the photoacoustic feedback signal. Imaging resolution improvement by scanning the object Next, we demonstrate the resolution improvement by imaging a black alpaca hair (25 μm diameter) placed behind an optical scatterer. To understand the nature of the resolution improvement, we perform photoacoustic imaging by scanning the hair under three different optical fields (uniform, random speckle and optimized speckle). A photoacoustic image of the hair illuminated with a uniform optical field is shown in Fig. 3a . Here the measured photoacoustic FWHM of the hair is found to be on average 79 μm, which agrees with the expected size given the acoustic resolution (see Supplementary Note 1 and Supplementary Fig. 2 ). With a glass diffuser placed in the optical path a random optical speckle field is created. The photoacoustic image reconstructed with this illumination is shown in Fig. 3b . Interestingly, the FWHM of the hair decreases to an average of 55 μm. The photoacoustic image from the random optical speckle field does show a resolution improvement, likely due to the speckle arrangement within the transducer (that is, a few intense speckles that provided improved resolution). Through genetic algorithm optimization of the optical wavefront on a large (43 μm diameter) alpaca hair the photoacoustic signal is enhanced by six. Photoacoustic imaging with the optimized wavefront provides both the highest SNR and the best resolution as shown in Fig. 3c . The measured FWHM of the alpaca hair decreases to 30 μm. Assuming the optimization creates an optical focus of similar size to that of Fig. 2c , the resolution increases by five to six times compared with the acoustic resolution. 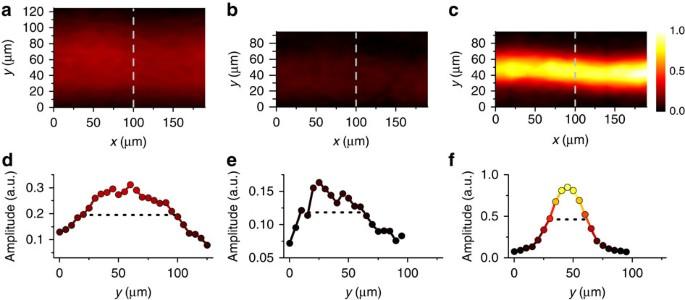Figure 3: Resolution measurement with 25-μm black alpaca hair. The photoacoustic images created with different optical illuminations: (a) acoustic resolution using uniform illumination (no scatterer), (b) random optical speckle field from scatterer, (c) wavefront optimized speckle focus. (d,eandf) show cross sections corresponding to the white dashed lines. Figure 3: Resolution measurement with 25-μm black alpaca hair. The photoacoustic images created with different optical illuminations: ( a ) acoustic resolution using uniform illumination (no scatterer), ( b ) random optical speckle field from scatterer, ( c ) wavefront optimized speckle focus. ( d , e and f ) show cross sections corresponding to the white dashed lines. Full size image Super-resolution photoacoustic imaging performed on a sweat bee wing, which provides an interesting complex structure, reveals significant resolution and signal improvement. As with the alpaca hair, we present photoacoustic images of the wing with uniform ( Fig. 4a ) and random speckle ( Fig. 4b ) optical illuminations for comparison. For the wavefront optimization we select an extended feedback region ( ∼ 40 × 40 μm) at the intersection of the large vein on the leading edge of the wing and a branching vein. After optimization the signal strength improved by a factor of 10 over the random speckle field illumination. We image the bee wing by scanning it behind the scatterer ( Fig. 4c ). The photoacoustic image significantly improves after optimization both in lateral resolution and SNR, which facilitates image reconstruction by sectioning the photoacoustic waveform temporally [18] ( Fig. 4d ). With the uniform and random speckle fields small features, visible in the optical image ( Fig. 4e ), such as hairs spaced 15–30 μm apart on the wing, result in a high background signal and broadening of the prominent vein features. However, with the optimized focus image, the hairs are individually resolved (see Supplementary Note 2 and Supplementary Fig. 3 ). By treating the 4 μm wide hairs as point sources we measure the optical resolution to be 13.2 μm through autocorrelation of the imaged hairs. 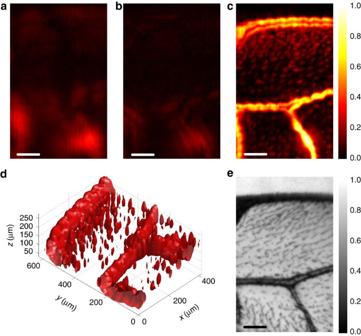Figure 4: Photoacoustic image reconstructions of sweat bee wing. The photoacoustic images created with different optical illuminations, scale bar, 100 μm: (a) acoustic resolution using uniform illumination (no scatterer), (b) random optical speckle field from scatterer, (c) wavefront optimized speckle focus. (d) Three-dimensional reconstruction of the optimized wavefront image, seeSupplementary Informationfor movie rendering. (e) The optical image of the same section of wing. Figure 4: Photoacoustic image reconstructions of sweat bee wing. The photoacoustic images created with different optical illuminations, scale bar, 100 μm: ( a ) acoustic resolution using uniform illumination (no scatterer), ( b ) random optical speckle field from scatterer, ( c ) wavefront optimized speckle focus. ( d ) Three-dimensional reconstruction of the optimized wavefront image, see Supplementary Information for movie rendering. ( e ) The optical image of the same section of wing. Full size image Imaging resolution improvement by scanning the transducer In applications involving imaging inside or through turbid media, one rarely has the ability to scan an object through a single focused point. In the more general case, the transducer focus is scanned and the wavefront optimized at each transducer focus position; thereby building an image point-by-point. In the previous experiments, the wavefront was optimized on a uniform, extended absorber and the spatial sensitivity of the transducer lead to a preferred optical focus at the centre of the acoustic focus after genetic algorithm optimization. If the wavefront is not optimized on an extended absorber, then the optimization routine will produce an optical focus at the position within the transducer focal region that produces the largest measured photoacoustic response. This response, in turn, depends on both the absorbed optical energy distribution and transducer point spread function [22] . As the transducer is scanned to build up a photoacoustic image, one does not know a priori the exact location of the focus at each step. Nevertheless, an optical focus is produced which moves from absorber to absorber to maximize the photoacoustic response while delivering significant spatial information ( Fig. 5a ) (see Supplementary Methods for details of the non-linear dispersive model that describes this system). Here we consider a simple one-dimensional scan across a resolution target consisting of 55±3-μm wide chromium bars separated by 55±3 μm ( Fig. 5b ). We first simulate the photoacoustic response to uniform and optimized illumination fields as the transducer is scanned across the target. The results ( Fig. 5c ) indicate that the optimized focus improves the ability to resolve the individual bars; a direct result of having a tight focus that seeks the strongest absorber rather than a response integrated over the entire focal volume. The experimental results ( Fig. 5d ) show good agreement with theory, with the optimized wavefront producing an enhanced photoacoustic response and allowing for the individual bars to be resolved; a result not possible using conventional (uniform or speckle field illumination) photoacoustics. In this case, the magnitude of the 50 MHz component of the photoacoustic signal was used for feedback in the optimization routine, giving an effective acoustic focal diameter (−6 dB) of 61 μm. The frequency spectra of the photoacoustic signals measured under uniform and random illumination show a central peak closer to 40 MHz and this peak evolves towards higher frequencies through the optimization process. To determine if the resolution obtained using the optimized wavefront exceeds the acoustic resolution at the frequency used for feedback, we band-pass filtered the photoacoustic responses under all illumination conditions about a central frequency of 50 MHz (See Supplementary Fig. 4 for the resulting response in this case). The improved resolution observed for the optimized wavefront remains, albeit at slightly reduced contrast (See Supplementary Fig. 4 ). Hence, we conclude the improved resolution is the result of a narrower spatial point spread function. 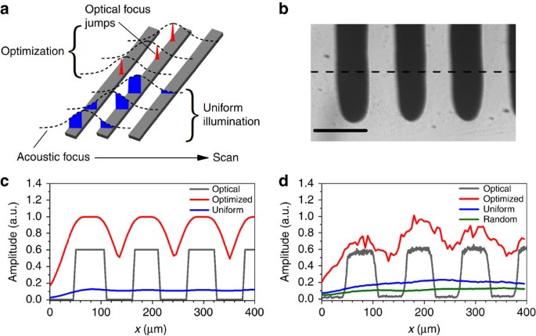Figure 5: Photoacoustic 1D scan. Photoacoustic image reconstructions of resolution bars by scanning the transducer. (a) Sketch showing the position of an optimized focus as the transducer scans the sample compared with the photoacoustic signal from uniform illumination. (b) Simulated one-dimensional (1D) scan comparing optimized focus to uniform illumination photoacoustic imaging. (c) Optical image of the sample. (d) Experimental photoacoustic 1D scan comparing uniform, random and optimized illuminations. scale bar, 100 μm. Figure 5: Photoacoustic 1D scan. Photoacoustic image reconstructions of resolution bars by scanning the transducer. ( a ) Sketch showing the position of an optimized focus as the transducer scans the sample compared with the photoacoustic signal from uniform illumination. ( b ) Simulated one-dimensional (1D) scan comparing optimized focus to uniform illumination photoacoustic imaging. ( c ) Optical image of the sample. ( d ) Experimental photoacoustic 1D scan comparing uniform, random and optimized illuminations. scale bar, 100 μm. Full size image In conclusion, we have proposed and demonstrated a technique to create an optical focus behind a scattering medium that enables improved resolution and SNR of photoacoustic imaging. The spatially varying feedback signal provided by the ultrasound transducer allowed the wavefront to evolve into a single speckle optical focus through mode competition. The method created an optical focal spot five times smaller than the acoustic focal spot size even though the optimization takes place on an extended absorber. The formation of this focus allowed for imaging absorbing samples at a higher resolution and SNR than possible with conventional techniques. Interestingly, the approach does not require use of the so-called memory effect [9] , [11] which would limit the applicability to weak or thin scatterers. The technique is thus ideal for imaging through an opaque wall with resolution beyond that provided by the feedback mechanism. Expanding this work for focusing inside biological tissue presents a significant challenge worthy of future investigation. In this work, we use an optical speckle grain size of 13 μm, which is large compared with the speckle grain size inside of a scattering biological sample ( ∼ λ/2). However, simulations indicate that as the ratio between the acoustic focus and the optical speckle size increases, a focus of a few speckles can still be created by increasing the number of the input modes and genetic algorithm iterations. The acoustic feedback volume may be constrained by utilizing a large numerical aperture detection transducer with a high centre frequency, along with time gating the photoacoustic response. In addition, non-linear photoacoustic feedback [23] provides another pathway towards focus optimization with decreasing speckle size. Wavefront optimization took ∼ 15 min per point in this work, limited by the 20-Hz repetition rate of the laser. Further improvements could be realized with a high repetition rate pulsed laser (taking care to limit the energy deposition to avoid deleterious heating effects) and digital micromirror device as a wavefront shaper [24] to drastically reduce the optimization time. The experimental data are obtained using the set-up illustrated in Fig. 2a . A collimated 532 nm, 5-ns pulsed laser (Continuum Surelight I20, 20-Hz repetition rate) illuminates a SLM (Boulder Non-linear Systems, 512 × 512 pixels) for wavefront shaping. The illuminated area of the SLM is 0.47 cm 2 and the corresponding optical fluence measured after the SLM is 9.4 μJ cm −2 . The SLM is imaged onto the back aperture of a long working distance microscope objective (× 5, 0.14 NA). The wavefront focuses into a water tank and onto the surface of a glass diffuser. An absorbing sample approximately 8 mm behind the glass diffuser is mounted onto a two-dimensional translation stage for scanning in the x and y dimensions using 5-μm step size. A 90 MHz (Olympus, V3512, 50 MHz bandwidth, 0.25 inch diameter, 0.5 inch. focal length) focusing ultrasound transducer placed in the water detects the photoacoustic signal. After pre-amplification, an oscilloscope records, digitizes and sends the detected signal to a computer for analysis. A one-dimensional translation stage is used for scanning the transducer in the second imaging modality where the wavefront is optimized for each position. To analyse the optical field, an Air Force resolution target is placed above the alpaca hair. Before ( Fig. 2b ) and after ( Fig. 2c ) wavefront optimization the reflecting target is lowered into the focus to deflect the light to an imaging lens such that the optical intensity distribution at photoacoustic imaging plane is imaged on the charge-coupled device. The resolution target also provides calibration for the system magnification. The refraction at the water tank wall produced astigmatism in the optical system that creates an image distorted in the y direction. For that reason, the FWHM is only measured in the x direction. The optical speckle size at the transducer focal plane for the random optical illumination and optimized wavefront cases were the same. The speckle illumination is created by encoding a flat phase on the SLM. For uniform optical illumination the scatterer is removed from the optical beam path ( Fig. 3a and Fig. 4a ). During wavefront optimization low frequency signals are removed using a second order Butterworth digital high-pass filter with an 80 MHz cutoff frequency to limit the feedback area. The highest cutoff frequency that could be used for the high-pass filter while maintaining sufficient signal-to-noise ratio for consistent wavefront optimization was 80 MHz. In contrast, image reconstructions do not use the high-pass filter, but instead use the unfiltered signal. These images are reconstructed with the maximum peak to peak value from the waveform from each position. To image the resolution target, wavefront optimization was achieved by maximizing the magnitude of the photoacoustic response at 50 MHz. This was close to the central frequency of the photoacoustic response subsequent to optimization and resulted in consistent values for the enhancement factor. How to cite this article : Conkey, D. B. et al . Super-resolution photoacoustic imaging through a scattering wall. Nat. Commun. 6:7902 doi: 10.1038/ncomms8902 (2015).